An information-theoretic principle implies that any discrete physical theory is classical It has been suggested that nature could be discrete in the sense that the underlying state space of a physical system has only a finite number of pure states. Here we present a strong physical argument for the quantum theoretical property that every state space has infinitely many pure states. We propose a simple physical postulate that dictates that the only possible discrete theory is classical theory. More specifically, we postulate that no information gain implies no disturbance or, read in the contrapositive, that disturbance leads to some form of information gain. Furthermore, we show that non-classical discrete theories are still ruled out even if we relax the postulate to hold only approximately in the sense that no information gain only causes a small amount of disturbance. Our postulate also rules out popular generalizations such as the Popescu–Rohrlich-box that allows non-local correlations beyond the limits of quantum theory. In contrast to classical theory, quantum theory has the remarkable property that the state space of every system has continuously many pure states. These are states that can be seen as states of maximal knowledge: they cannot be prepared by flipping a (possibly biased) coin to decide between two different preparation procedures to be executed, hiding the outcome of the coin flip. Even the qubit, the smallest possible system with no more than two perfectly distinguishable states, has continuously many such states. This non-discreteness of quantum theory contrasts sharply with classical theory, where systems with a finite number of perfectly distinguishable states have the same finite number of pure states. While from a mathematical point of view, this quantum property is satisfactorily explained as a consequence of the mathematical framework of quantum theory, a physical explanation of this phenomenon is less evident. Indeed, one might conjecture that the actual state space of a physical system really was discrete with only finitely many pure states ( Fig. 1 ) [1] , [2] . The fact that experiments have not found a deviation from the continuous nature of the quantum state spaces could then be explained by insufficient measurement precision. A qubit, for example, could be described by a polytope that approximates the continuous spherical shape of the Bloch ball very well, while it actually is a discrete system. Quantum gravitational considerations have led some authors to the idea that indications for the discreteness of spacetime could in turn provide an indication for the discreteness of quantum state spaces [1] , [2] . Such considerations might suggest state spaces with an extremely high number of pure states, but as long as the number of pure states is finite, they would differ from quantum state spaces in a fundamental way. 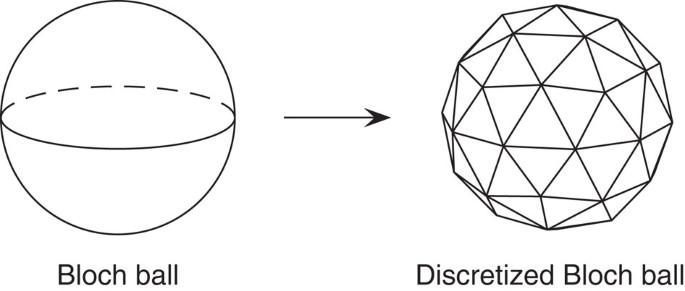Figure 1: Illustration of discretized state spaces. One might conjecture that physical state spaces are discrete in the sense that they only have a finite number of pure statesIn such discrete state spaces, the pure states are given by the corners of the state space. Figure 1: Illustration of discretized state spaces. One might conjecture that physical state spaces are discrete in the sense that they only have a finite number of pure statesIn such discrete state spaces, the pure states are given by the corners of the state space. Full size image In this work, we present a strong physical counter-argument to the idea that quantum theory could be replaced by a theory with discrete state spaces. This argument is derived from a postulate that claims a very basic principle for measurements. It states that every (pure) measurement can be performed in a way such that the states with a definite outcome (that is, the states with an outcome of probability one) are left invariant. We regard this principle to be a natural property of a theory that describes physical measurements, so we impose it as a postulate. Performing a measurement with a definite outcome does not give any information, while performing a measurement for which the outcome is not known in advance can be seen as a process of gaining information. This allows to regard our postulate as a converse to the well-known fact in quantum theory that information gain causes disturbance [3] : we postulate that a measurement with no information gain causes no disturbance. We prove that a non-classical probabilistic theory that satisfies this postulate cannot be discrete. By a discrete system, we mean a system for which the state space has only finitely many pure states. In other words, we show that every theory that satisfies our postulate must either be classical or it must have infinitely many pure states. The framework We formulate our result in the abstract state space framework [4] , [5] , [6] , [7] . This framework arises from the idea to consider the largest possible class of physical theories (more precisely, generalized probabilistic theories) which satisfy minimal assumptions, containing classical and quantum theory as special cases. This allows us to study properties of quantum theory, like the non-discreteness of the state space, from an outside perspective. Here, we discuss these minimal assumptions very briefly and refer to Pfister [8] for a detailed introduction to the abstract state space framework and its mathematical background. The framework, which relies on four minimal assumptions, is based on the idea that any physical theory admits the notions of states and measurements. Their interpretation is assumed to be given. The first assumption is that the normalized states form a convex subset of a real vector space A . The underlying motivation is the idea of probabilistic state preparation: if are states that can each be prepared by a corresponding preparation procedure, then executing the preparation procedures with probability p and 1− p should also lead to a state (described by the convex sum ), which should therefore be an element of as well. The second assumption is that the dimension of the vector space containing the set of states is arbitrarily large but finite. This is a purely technical assumption intended to make the involved mathematics feasible. The third assumption is that the set of states is compact. Although there might be some physical motivation for this assumption, we shall be satisfied with considering it as a technical assumption. Before we discuss the fourth assumption, we make a few comments on the structure of . The extreme points of are the pure states of the system, the other elements are called mixed states. As is a convex and compact subset of a finite-dimensional vector space A , every element of is a convex combination of the extreme points of (ref. 9 ). Thus, every state is a convex combination of pure states. As a convex combination is a sum with positive weights that sum up to one, a state can be seen as a probability distribution over pure states. In general, this probability distribution is not unique. In classical theory, however, it is (see the example below). In addition to the normalized states , an abstract state space A also contains the subnormalized states , which are given by all rescalings of the normalized states by factors between zero and one. The fourth assumption states, roughly speaking, that every mathematically well-defined measurement is regarded as a valid measurement: a measurement is a finite set ={ f 1 ,…, f n } of functions that are called effects, each corresponding to an outcome of the measurement. For a state , the value is interpreted to be the probability that the measurement yields the outcome i when the system was in the state before the measurement. Thus, one must have for all . If the measured system was in the state with probability p and in the state with probability 1− p , then the probability of getting the outcome has to be identical to as is regarded to be a state in its own right (in accordance with the first assumption). Skipping a few details, this means that effects are assumed to be linear. Moreover, the effects of a measurement have to sum up to the so-called unit effect for which for all (as the probability that any outcome occurs has to be one). The fourth assumption is that every set of such linear functionals (effects) is a valid measurement. We denote the set of all effects on an abstract state space by , and we denote measurements (that is, sets of effects that sum up to the unit effect) by calligraphic letters ( M or N in this paper). We would like to emphasize that the fourth assumption, which connects the geometry of the states with the geometry of the effects [8] , is standard but non-trivial and of crucial technical importance for our result. A compelling physical motivation does not seem to be obvious, so it should be regarded as a tentative assumption on the way to a better understanding of quantum theory. Note that as a consequence of this assumption, a theory where the set of states is a quantum state space but where the measurements are restricted to a proper subset of the positive operator valued measures (POVMs) is not part of the framework (c.f. quantum theory in the examples below). In quantum information science, it is always assumed that the full set of POVMs can be performed. These four assumptions determine the framework of abstract state spaces. This structure is sufficient as long as one is only interested in measurement statistics of one-shot measurements. If one wants to describe several consecutive measurements, one has to introduce measurement transformations. We will discuss this below, but first, we make a few examples. In the following, we introduce a few examples of theories that can be formulated in the abstract state space framework. (More examples can be found in [8] .) While quantum and classical theories are theories of actual physical significance, other theories that we introduce have the role of toy theories, which are helpful to understand the framework. Especially the square and the pentagon, which are instances of polygon models (see below), will serve as useful examples in the illustration of the proof idea of our result. As a first example, let us have a look at quantum theory. The set of states of a (finite-dimensional) quantum system is given by Ω A =() for some (finite-dimensional) Hilbert space , where () denotes the positive operators on with unit trace (the density operators). These operators form a compact convex subset of A= Herm(), the vector space of Hermitian operators on . Every quantum system has continuously many pure states. The most general description of measurement statistics in quantum theory is given by a POVM, which is a set of positive operators that sum up to the identity-operator I on . They give rise to the effects that sum up to the unit effect given by for all . In analogy to our comment above, we emphasize that a theory where the states form a proper subset of a quantum state space but where the measurements are given by not more than POVMs fails to satisfy the fourth assumption of the framework because a reduction of the allowed states requires an extension of the effects. Another example is classical theory. The states of a (finite) classical theory are given by a simplex, that is, by the convex hull of finitely many affinely independent points. (We say that points in a real vector space are affinely independent if no point is an affine combination of the other points, that is, if for every , there are no real coefficients with such that .) Examples of simplices are given by a line segment, a triangle, a tetrahedron, a pentachoron and so on. Every element of a simplex is a unique convex combination of the extreme points of ( Fig. 2 ). Thus, for a simplex , the states are in a one-to-one correspondence with the probability distributions over the pure states, which in the case of a simplex are perfectly distinguishable. This allows to interpret the pure states as classical symbols. In a classical system, there is a generic measurement. For a given state , the outcome probabilities for this measurement are precisely the coefficients in the convex sum of the pure states that yield . 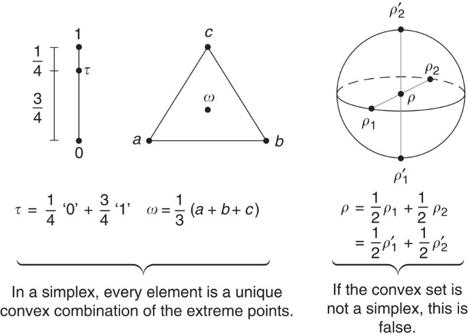Figure 2: (Non-)Uniqueness of convex decompositions. A classical system is described by a simplex, which has the property that every point is a unique convex combination of the extreme points. Thus, a state in a classical system corresponds to a unique probability distribution over classical symbols. Figure 2: (Non-)Uniqueness of convex decompositions. A classical system is described by a simplex, which has the property that every point is a unique convex combination of the extreme points. Thus, a state in a classical system corresponds to a unique probability distribution over classical symbols. Full size image A more general class of examples is given by what we call discrete theories. We say that is a discrete state space if it is the convex hull of finitely many (not necessarily affinely independent) points. As is compact, this is equivalent to saying that the theory has only finitely many pure states. Classical theory is an example of a discrete theory, while quantum theory is not. Very illustrative examples are given by the polygon models [10] : these are abstract state spaces where is a regular polygon, so they are special kinds of discrete theories. As the whole situation can be drawn in only three dimensions, the polygon models provide examples for which we can give a picture ( Fig. 3 ). To see the interplay of states and effects in such a low-dimensional example, it is useful to represent effects as vectors in the same space as the states [10] . To evaluate an effect at some state, one simply takes the scalar product of the state and the vector representing the effect. In the Methods section below, the square and the pentagon will be the central examples in the illustration of the proof idea. 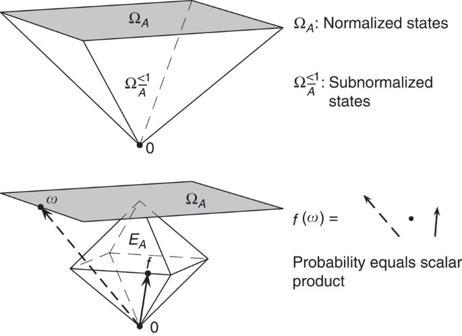Figure 3: The square polygon model. The upper part of the figure shows the set of normalized states(grey), together with the subnormalized states(white ‘pyramid’), which are given by all rescalings of normalized states with factors between zero and one. In the lower part of the figure, the subnormalized states are omitted. Instead, the effectsEAare shown (here they correspond to an octahedron). The reader who is familiar with the mathematics of ordered vector spaces may notice that the effects arise from the structure of the dual cone(more precisely, the effects form an order interval [0,uA] inA)8. Here, they are represented as vectors in the same space as the states. To calculate a probability, one simply takes the scalar product of the vectorand the vector representingf. Figure 3: The square polygon model. The upper part of the figure shows the set of normalized states (grey), together with the subnormalized states (white ‘pyramid’), which are given by all rescalings of normalized states with factors between zero and one. In the lower part of the figure, the subnormalized states are omitted. Instead, the effects E A are shown (here they correspond to an octahedron). The reader who is familiar with the mathematics of ordered vector spaces may notice that the effects arise from the structure of the dual cone (more precisely, the effects form an order interval [0, u A ] in A ) [8] . Here, they are represented as vectors in the same space as the states. To calculate a probability , one simply takes the scalar product of the vector and the vector representing f . Full size image So far, we have discussed the core structure of abstract state spaces: states and effects. They only allow for the description of one-shot measurement statistics. If one wants to describe the statistics of several consecutive measurements, then one has to specify what happens to the state of the system when a measurement is performed (otherwise, the statistics of the subsequent measurement cannot be described). In other words, one has to specify a rule for post-measurement states. The structure of an abstract state space, however, does not provide such a rule and leaves open the question of how to specify post-measurement states. We deal with this question and consider some extra structure on abstract state spaces that provides a rule for post-measurement states. We describe the transition from the initial state of the system (before the measurement) to the post-measurement state by what we call a measurement transformation. Such transformations have been considered, for example, in [11] , [12] , [13] . We go one step further. Our result makes a statement about the existence of measurement transformations in abstract state spaces that satisfy a certain postulate. As we have just mentioned above, the general idea is that a measurement transformation specifies a rule for how post-measurement states are assigned. However, in a physical theory, how such a rule looks like depends on the particular situation that one wants to describe. To be more specific, we can think of at least three such situations (we will make quantum examples below), which correspond to the case where (a) the observer finds out the outcome of the measurement and describes the state of the system after the measurement conditioned on that outcome; (b) the observer describes the system after the measurement by a subnormalized state for the hypothetical case that a particular outcome occurred, incorporating the probability of that outcome into the post-measurement state; and (c) the observer does not find out the outcome of the measurement and describes the state of the system after the measurement, knowing only that the measurement has been performed. A physical theory has to allow for a mathematical description for all of these cases. Each of the three situations can be described by a particular kind of map. To understand the difference between them, it is helpful to see how these maps look like for the particular case of quantum theory. There, if the measurement is a projective measurement , the maps are given by Lüders projections [14] (the literature is ambiguous about which of the three maps is called a Lüders projection, but as they are very closely related, this usually does not lead to problems). The situations (a), (b) and (c) above are described by the following maps: in situation (a), if the outcome associated with projector P k is measured, then the state is transformed as In situation (b), considering the outcome associated with projector P k , the state transforms into a subnormalized state as In situation (c), if the outcome of the measurement is unknown, the state is transformed as Most introductory textbooks on quantum theory only discuss situation (a). Note that (a) is not a linear map. By the definition that we will make below, it should not be called a transformation. The maps (b) and (c) are linear. The map (b) describes what Lüders calls a ‘measurement followed by selection’, whereas the map (c) describes what he calls a ‘measurement followed by aggregation’ [14] . The preceding discussion allows us to understand what we mean by a measurement transformation. By a measurement transformation, we mean a map of type (b). Note that such a map leads to subnormalized post-measurement states rather than normalized ones. The norm of the post-measurement state (the trace-norm in the quantum case, ) is equal to the probability that the outcome occurs (which is what we mean by ‘the probability of that outcome is incorporated into the state’). Choosing maps of type (b) (rather than maps of type (a) or (c)) as the subject matter is not a relevant restriction as the three types of maps are so closely related that insights into one of these maps translate into insights into the other maps as well. In particular, from the map of type (b), one can construct the map of type (a) by rescaling the images with the inverse probability and the map of type (c) by summing up over all outcomes. With the above motivation in mind, we now proceed to the task of formally defining what we mean by a measurement transformation on an abstract state space. A transformation T on an abstract state space A is a linear map T : A → A such that . The motivation for the linearity of transformations is similar to the motivation for the linearity of effects. The linearity expresses a compatibility condition for probabilistically prepared states: if the system is in a state with probability p and in a state with probability before the transformation, then the transformed state has to coincide with as is regarded as a state in its own right. (A more rigorous argument would require for all effects f , which eventually boils down to what we have just required.) A measurement transformation has to satisfy one more condition. As we have explained above, a measurement transformation is associated with a particular outcome, or more precisely, with a particular effect. If T is a measurement transformation for an effect f , then we require that the norm of the transformed state is equal to the probability for measuring the outcome associated with f . In short, we require In quantum theory, where u A is given by the trace, this property is satisfied for projective measurements as the Lüders projection gives . We will only consider measurement transformations for a special class of effects that we call pure effects. We say that an effect is pure if it is an extreme point of the (convex) set of effects E A , and we say that a measurement ={ f 1 ,…, f n } is pure if every effect is pure. It turns out that in the case of quantum theory, an effect of a POVM element F is pure if and only if F is a projector [8] . Thus, we only consider measurement transformations for a class of effects that, in the case of quantum theory, reduces to projectors. For this class, the measurement transformations are given by Lüders projections. The fact that we will restrict our considerations to pure effects is not a restriction of the validity of our result. Quite the contrary, this makes our result stronger. As we will see below, our postulate claims a property of measurement transformations for pure effects rather than claiming this property for all effects. This results in a weaker postulate, so every implication derived from this postulate leads to a stronger result. As we will see later, we will restrict the claim of the postulate to an even smaller subclass of effects (see the Methods section and the Supplementary Note 1 for further details). In a nutshell, a measurement transformation for a pure effect f is a linear map T : A → A with and . The postulate Before we can formulate our result, we first state our postulate. For a mathematically precise formulation, we refer to the Methods section and the Supplementary Note 1 of this article. The postulate reads: Every pure measurement can be performed in a way such that the states for which it yields a certain outcome (that is, the states with an outcome of probability one) are left invariant. In more illustrative terms, this can be rephrased by saying that no information gain implies no disturbance. In more technical terms, the postulate states that for every pure effect , there exists an associated measurement transformation T with such that for all states with , we have that . The existence of such a measurement transformation T is what is meant by saying that there exists a way to perform the measurement. Furthermore, note that without looking at the definition of a measurement transformation, saying that ‘there exists a way to perform the measurement’ may appear trivial by itself. After all, doing nothing and outputting the measurement outcome (associated with) f preserves and yields f with probability 1. This case is ruled out by the definition of a measurement transformation. More precisely, note that T must be such that for all states . That is, it yields the correct probabilities for any state that we wish to measure. It is interesting to note that the actual proof of our main result only needs an even weaker but rather technical requirement (see the Methods section). To see the link to information gain, note that the Shannon information content (see, for example, [15] ) is zero for any outcome of an experiment that occurs with certainty. As such, is equivalent to stating that no information gain occurs. The demand that says that the state is unchanged, that is, no disturbance has occurred. Quantum theory and classical theory satisfy this postulate. In quantum theory, for example, if a system is in a state such that a projective measurement has some outcome k with probability , then the transformation leaves the state invariant. Quantum theory even satisfies the postulate in a much stronger form in the sense that little information gain also causes only little disturbance. This can be seen from a special case of the gentle measurement lemma [16] , [17] . It states that if measuring an outcome associated with a projector F has probability , then measuring that outcome disturbes the state by no more than . Setting , this reduces to our postulate. However, we emphasize that our postulate is much weaker than postulating the gentle measurement lemma. We also note that our postulate does not make any assumptions about locality, that is, it does not make a statement about whether verification measurements of bipartite states can be implemented on local quantum systems or locally disturb the state as has been considered in Popescu and Vaidman [18] . Even though the statement of the postulate is very concise, it may appear unsatisfying as it involves the abstract concept of a state, which is something that one cannot observe directly. However, it can be reformulated in purely operational terms, referring only to directly observable objects, namely measurement statistics. Such a reformulation is possible because two states can be regarded as being identical if and only if they induce the same measurement statistics for every measurement (in more mathematical terms, a state is an equivalence class under the relation for all ) [19] . Hence, instead of making statements about states, one can make statements about the statistics of all potential measurements. 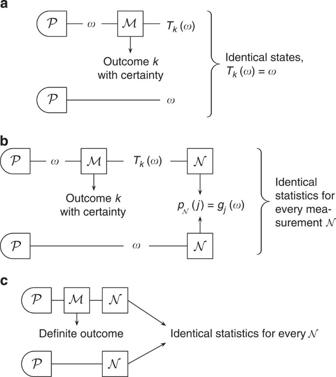Figure 4: A reformulation of the postulate in purely operational terms. Instead of referring to initial and post-measurement states, the reformulated version states that a measurement with a definite outcome does not influence the statistics of any subsequent measurement, so it only refers to directly observable quantities. This reformulation can be understood as follows: consider a preparation that outputs an initial stateand a measurement ={f1,…,fn} such thatfor somek. According to the postulate, the state of the system after the two experiments shown in (a) are identical. Thus, if the two experiments are followed by any measurement, say ={g1,…,gl}, then the statistics of the -measurement coincide (see part (b) of the figure). The -statistics coincide for every measurement . This is equivalent to saying that the states before the -measurement (that is,and) are identical. Thus, we do not need to refer to states and can reformulate the postulate as: if a measurement has a definite outcome, then performing this measurement does not influence the statistics of any subsequent measurement. This is shown diagrammatically in part (c) of the figure. Figure 4 illustrates the idea of this reformulation. Figure 4: A reformulation of the postulate in purely operational terms. Instead of referring to initial and post-measurement states, the reformulated version states that a measurement with a definite outcome does not influence the statistics of any subsequent measurement, so it only refers to directly observable quantities. This reformulation can be understood as follows: consider a preparation that outputs an initial state and a measurement ={ f 1 ,…, f n } such that for some k . According to the postulate, the state of the system after the two experiments shown in ( a ) are identical. Thus, if the two experiments are followed by any measurement, say ={ g 1 ,…, g l }, then the statistics of the -measurement coincide (see part ( b ) of the figure). The -statistics coincide for every measurement . This is equivalent to saying that the states before the -measurement (that is, and ) are identical. Thus, we do not need to refer to states and can reformulate the postulate as: if a measurement has a definite outcome, then performing this measurement does not influence the statistics of any subsequent measurement. This is shown diagrammatically in part ( c ) of the figure. Full size image Main findings In terms of the postulate, our result can now be stated as follows: an abstract state space that satisfies the postulate is either non-discrete (that is, it has infinitely many pure states) or it is classical. This means that if a physical system is described by an abstract state space where the set of states is a polytope that is not a simplex (that is, if it is a discrete non-classical system), then it violates our postulate. Furthermore, our result is robust in the sense that discrete non-classical theories are ruled out even if the postulate is weakened to an approximate version. To formulate this approximate version of the result, we assume that A is equipped with a norm . This induces a distance function on A . We prove that for every discrete non-classical theory, equipped with some norm , there is a positive number such that the implication (where T is the measurement transformation for f ) cannot be satisfied for every pure effect . We prove this approximate case, which is a stronger version of the result, in the Supplementary Note 2 . Our simple postulate rules out discrete non-classical theories, while classical and quantum theory satisfy the postulate. Read in the contrapositive, our postulate says that disturbance implies information gain. Any theory that does not satisfy our postulate thus allows for disturbance without a corresponding ability of information gain. Note that even in a theory that a priori only defines transformations T , one can define effects as . We also note that our postulate rules out several alternatives to quantum theory, most notably the famous Popescu–Rohrlich-box (PR-box) [20] , [21] , [22] that allows a violation of the CHSH inequality [23] far beyond the limits of quantum theory. More specifically, the PR-box achieves the algebraically maximal violation of the CHSH inequality, while still respecting the law that no information can travel faster than light. This is in spirit similar to other approaches such as information causality [24] , communication complexity assumptions [25] , the assumption of local quantum mechanics [26] or the uncertainty principle [27] . We emphasize, however, that whereas this is a nice byproduct of our result, our real aim lies in the study of local physical systems with the goal to identify just one postulate that sheds light on the simple question whether the state space should be discrete or continuous. It is very satisfying that this question can be understood by introducing just a single postulate. One may wonder whether our postulate does in fact rule out all theories but classical and quantum mechanics. To answer this question, let us first be more precise about what we mean by ‘a theory is (not) ruled out by the postulate’. We mentioned in the preceding section that for general abstract state spaces, measurement transformations are not specified, so we cannot make statements saying that the (unique) measurement transformations do (not) satisfy our postulate. Instead, we can discuss the following well-defined question: given an abstract state space, is it true that for every pure effect, there exists a measurement transformation that satisfies our postulate? If this is the case, then we say that the theory can satisfy the postulate, or that it is not ruled out by the postulate. If this is not true, then we say that the theory cannot satisfy the postulate, or that it is ruled out by the postulate. This is the precise meaning of our statement that ‘discrete non-classical theories are ruled out by the postulate’. Using this terminology, we can identify a class of theories that, in addition to classical and quantum theory, is not ruled out by the postulate: the strictly convex theories can satisfy our postulate. These are theories where the set of normalized states is strictly convex, that is, the boundary contains no line segment. There are more theories that can satisfy the postulate, but we do not know a concise classification. For example, a state space formed like a piece of pizza is ruled out by the postulate, while a state space formed like an ice cream cone is not. 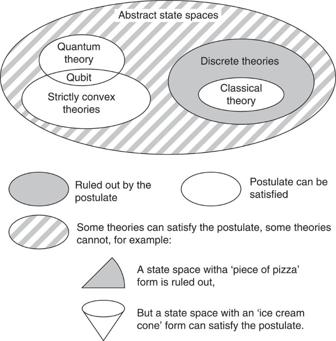Figure 5: An overview over the abstract state spaces ruled out by the postulate.  Figure 5 gives an overview. Figure 5: An overview over the abstract state spaces ruled out by the postulate. Full size image In the recent past, there have been several attempts to derive (finite-dimensional) quantum theory within a framework of probabilistic theories [12] , [28] , [29] . The idea is the following. One starts with a very general framework of probabilistic theories (like the abstract state space formalism). Then, one imposes a few physical postulates (our postulate can be seen as one such postulate). If one manages to show that all theories in this framework other than quantum theory are ruled out by these physical postulates, then this can be seen as a physical derivation of quantum theory. As our postulate rules out quite a large fraction of all possible abstract state spaces already ( Fig. 5 ), it seems promising that adding just a few more postulates might be sufficient to rule out all theories except for quantum theory. However, we do not make such an attempt and focus on one particular aspect only, introducing only one postulate. What makes our postulate special is that its nature is very different from the postulates that have been considered in this context so far. Many approaches focus on the aspect of non-locality, introducing rules for how physical systems are combined to form bi- or multi-partite systems. In contrast, our approach deals with local state spaces only, making a statement about post-measurement states. Within probabilistic theories, this aspect has gained less attention in the literature so far. The fact that, within the framework of abstract state spaces, we introduce just one postulate (instead of a set of postulates) helps us to understand its influence on one particular aspect of physical theories. One might argue that an experimental proof of the non-discreteness of physical state spaces needs infinite measurement precision as the verification of the postulate that (strict equality) requires the verification that and give rise to the same measurement statistics (to arbitrary precision). Hence, our result is experimentally less accessible than other no-go theorems (for example, the Bell Inequality, where it is sufficient to verify the violation of a single statistical inequality). There is a partial reply to this objection. As we have mentioned before, there is an approximate version of our result. It states that for a given polytope P , there is a positive number such that the postulate can be weakened to the following form (without changing the validity of the result): if a measurement on a state has an outcome with probability one, then performing the measurement does not change the state of the system by more than (for details, see the Supplementary Note 2 ). Thus, even if one weakens the postulate to allow for an -disturbance of the state, it still rules out the polytope P . This is a stronger form of the result. It states that in order to rule out a given polytope experimentally, only finite measurement precision is needed (quantified by ). However, the allowed disturbance depends on the polytope P , so in order to rule out all polytopes experimentally, infinite measurement precision is needed because for every measurement error, there could be a polytopic theory for the measured system for which the allowed disturbance is too small to be tested. Overview In this section, we sketch the idea of the proof of our main result. This will lead to geometric pictures that illustrate the incompatibility of non-classical discrete state spaces with our postulate ( Fig. 6 and Fig. 7 ). For the full version of the proof and for a proof of the approximate version of our result, see the Supplementary Notes 1 and 2 of this article, respectively. 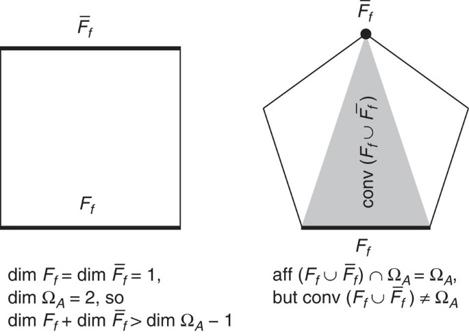Figure 6: Violation of the conditions stated in the lemma. The square and the pentagon serve as very basic examples of abstract state spaces that violate the conditions stated in the lemma. The square violates condition (a), while the pentagon violates (b). Figure 6: Violation of the conditions stated in the lemma. The square and the pentagon serve as very basic examples of abstract state spaces that violate the conditions stated in the lemma. The square violates condition (a), while the pentagon violates (b). 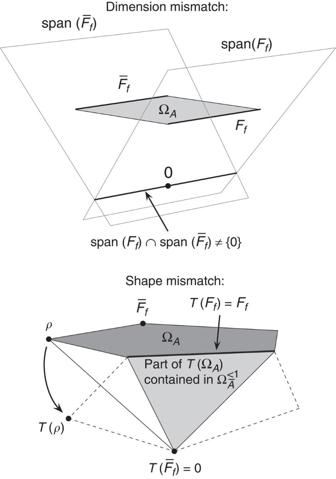Figure 7: Consequences of the violation of conditions (a) or (b). This figure illustrates geometrically why the square and the pentagon violate our postulate. Intuitively, all non-classical discrete state spaces exhibit either a dimension or a shape mismatch. Full size image Figure 7: Consequences of the violation of conditions (a) or (b). This figure illustrates geometrically why the square and the pentagon violate our postulate. Intuitively, all non-classical discrete state spaces exhibit either a dimension or a shape mismatch. Full size image Here, we aim for a geometric understanding of the proof. It is mainly based on a lemma that establishes geometric criteria for a set of states that is compatible with our postulate. To illustrate this lemma, we provide two very basic examples that violate these criteria: the square and the pentagon ( Fig. 6 ). For these two examples, it is easy to see geometrically why they cannot satisfy our postulate (as we will illustrate in Fig. 7 ). Finally, we describe roughly how we prove that every polytope that satisfies the conditions of the lemma is a simplex (which is our main result). Before we sketch the proof of the main result, it is useful to define in a bit more detail what an abstract state space is. For detailed definitions of the framework see the Supplementary Note 1 of this article, for a detailed motivation of the framework with detailed examples see Chapter 3 in Pfister [8] . The formal setup As illustrated in Fig. 8 , an abstract state space is fully specified by a tuple , where A is a real finite-dimensional vector space, A + is a cone in A and u A is a linear functional on A (called the unit effect). This linear functional is required to be strictly positive on the cone A + (that is, for all ). The tuple gives rise to the normalized states and the subnormalized states in the following way (c.f. Fig. 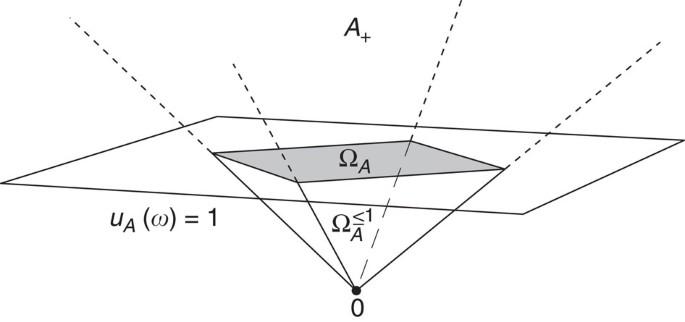Figure 8: Visualization of the state cone. The states of any normalization are given by a coneA+in the real vector spaceA. The linear functionaluAgives the normalization of a state, so the intersection ofA+with the plane described bygives the normalized states, while the subnormalized statesare those elements ofA+whereuAtakes values between 0 and 1. 8 ): Figure 8: Visualization of the state cone. The states of any normalization are given by a cone A + in the real vector space A . The linear functional u A gives the normalization of a state, so the intersection of A + with the plane described by gives the normalized states, while the subnormalized states are those elements of A + where u A takes values between 0 and 1. Full size image The set E A of effects on A is given by the linear functionals that take values between zero and one on the states , that is where A is the dual space of A . A measurement is given by a finite set of effects such that the effects sum up to the unit effect u A , that is, . Recall that if the system is in the state before the measurement described by ={ f 1 ,…, f n }, then the probability for outcome k is given by . As we have mentioned earlier, we restrict ourselves to pure effects when we deal with post-measurement states (that is, with measurement transformations). The pure effects are the extreme points of E A . A pure effect has the property that the set of states that have probability is a face of [8] . A face of is a convex subset with the property that every line segment whose endpoints are contained in F must be fully contained in F , that is, a face is some kind of ‘extreme subset’. For a pure effect f , this allows us to define the certain face F f of f by Analogously, the set of states that have probability is a face of as well [8] . We call it the impossible face of f and define it by The notion of the certain face and the impossible face of an effect is central in our proof. A transformation on an abstract state space is a linear map T : A → A that is positive (that is, T ( A + ) ⊆ A + ) and does not increase the norm of the states, that is, u A ( T ( ω ))≤ u A ( ω ) for all ω ∈ A + . Equivalently, a transformation is a linear map T : A → A with . Recall that we describe the state change due to a measurement by introducing measurement transformations. If a measurement yields an outcome associated to a pure effect f ∈ E A , then the transformation of the state is described by , where T is the measurement transformation for f . As mentioned, we require that T is a transformation that satisfies . With these definitions at hand, we can formulate our postulate as follows: for every pure effect f ∈ E A , there is a transformation T : A → A such that and T ( ω )= ω for every ω ∈ F f . Note that we only postulate the existence of a measurement transformation for f that satisfies our postulate. For the actual proof, we will require an even weaker condition. We will not require the existence of such a measurement transformation for every pure effect but only for pure effects for which the certain face F f is what we call a minus-face of . This is a face that is exactly one dimension smaller than . This weakening of the postulate is particularly useful for the proof of the approximate version of our result. Basic idea of the proof To derive the result, we first prove a lemma that establishes geometric criteria that a set of states has to satisfy to be compatible with our postulate. Given a pure effect f ∈ E A , the lemma tells us geometric criteria for the certain face F f and the impossible face of f , which are necessary for the existence of a measurement transformation satisfying our postulate. Let be an abstract state space and let f ∈ E A be a pure effect. If there exists a transformation T : A → A such that and T ( ω )= ω for every ω ∈ F f , then, (a) (b) where aff(·) and conv(·) denote the affine hull and the convex hull, respectively (the reader unfamiliar with these two notions is referred to the Supplementary Note 1 ). To get a geometric idea for the two conditions (a) and (b), it is useful to consider abstract state spaces that violate these conditions. The two simplest examples we can think of are the square and the pentagon, depicted in Fig. 6 . To see why the conditions (a) and (b) are necessary for the existence of a transformation compatible with our postulate, we now examine what goes wrong in the case where one of the conditions is violated. If condition (a) is violated, a contradiction occurs that we call a dimension mismatch. If (b) is violated, then we say that a shape mismatch occurs. Again, the square and the pentagon serve as good examples for a geometric illustration. We first look at the dimension mismatch. If condition (a) is violated (that is, ), then there is no linear map T such that In particular, there is no transformation with these two properties. To see this, there are two things to notice. First, equation (10) implies that for all (c.f. the definition (9) of ). As the zero-vector is the only state (that is, the only element of ) for which , it follows that the whole impossible face has to be mapped to the zero-vector. By the linearity of T , this implies that the restriction of T to is the zero-operator on : Second, the postulate (11) and the linearity of T imply that the restriction of T to is the identity-operator on : However, in the case where , equations (12) and (13) lead to a contradiction. In this case, the intersection is a subspace that is at least one-dimensional ( Fig. 7 ). Equations (12) and (13) imply that on this subspace, T has to be the zero-operator and the identity-operator simultaneously, which could only be satisfied if the subspace would be {0}. Now we look at the shape mismatch. If condition (b) is violated (that is, ), then for every linear map that satisfies equations (10) and (11), there is a state such that (that is, is not a state). Therefore, such a T cannot be a transformation. To see this geometrically, it is useful to consider the pentagon for a particular choice of the effect f where the certain face F f is an edge of the pentagon ( Fig. 7 ). Equation (10) implies that the impossible face is mapped to the zero-vector, while equation (11) means that the certain face F f is left invariant. In the case of the pentagon illustrated in Fig. 7 , there is precisely one linear map T with these two properties. It maps the normalized states (dark grey surface in the figure) to a set in the vector space (dashed lines) which is not contained in (the truncated cone between 0 and ). In particular, there is a such that . If one compares Fig. 7 with Fig. 6 , then one can see that the part of that is mapped to a subset of (light grey face in Fig. 7 ) is precisely given by (grey part in Fig. 6 ). However, the part of that is mapped outside of is given by (the white part in Fig. 6 ). This observation generalizes to statement (b) of the Lemma: if (a) is satisfied, then is contained in if and only if . These two examples illustrate all that can go wrong for discrete theories. We show that for every discrete theory (that is, for every theory where is a polytope), either condition (10) or (11) is violated (so either a dimension mismatch or a shape mismatch occurs), except for the case where is a simplex (that is, for classical theories). To show this, we proceed as follows. We consider an abstract state space ( A , A + , u A ) where is a polytope. We assume that for every pure effect for which the certain face F f is a minus-face of , there is a measurement transformation satisfying the postulate (11). In a first step, we show (using the lemma) that every polytope that is compatible with our postulate has a property that we call being uniformly pyramidal. This means that for every minus-face F of , it holds that there is a point such that (see the Supplementary Note 1 for more intuition). In a second step, we show that every uniformly pyramidal polytope is a simplex. This shows that every discrete theory satisfying our postulate has to be classical. How to cite this article: Pfister, C. & Wehener, S. An information-theoretic principle implies that any discrete physical theory is classical. Nat. Commun. 4:1851 doi: 10.1038/ncomms2821 (2013).